Amyloid-associated activity contributes to the severity and toxicity of a prion phenotype The self-assembly of alternative conformations of normal proteins into amyloid aggregates has been implicated in both the acquisition of new functions and in the appearance and progression of disease. However, while these amyloidogenic pathways are linked to the emergence of new phenotypes, numerous studies have uncoupled the accumulation of aggregates from their biological consequences, revealing currently underappreciated complexity in the determination of these traits. Here, to explore the molecular basis of protein-only phenotypes, we focused on the Saccharomyces cerevisiae Sup35/[ PSI + ] prion, which confers a translation termination defect and expression level-dependent toxicity in its amyloid form. Our studies reveal that aggregated Sup35 retains its normal function as a translation release factor. However, fluctuations in the composition and size of these complexes specifically alter the level of this aggregate-associated activity and thereby the severity and toxicity of the amyloid state. Thus, amyloid heterogeneity is a crucial contributor to protein-only phenotypes. Protein amyloids expand the range of phenotypes associated with a single genotype by serving as novel, self-replicating epigenetic determinants. In these cases, the heritable information is encoded by alternative protein conformations, which have the propensity to self-assemble into amyloid fibres. These complexes, in turn, associate with and incorporate other conformers of the same protein, effectively templating their refolding to the amyloidogenic state [1] , [2] . Through this process, the persistence, progression and transmission of a diverse array of phenotypes, ranging from neurodegenerative diseases in mammals to alternative gene expression states in yeast, becomes possible [1] . The link between amyloid assembly and its biological consequences varies by protein, but two general models have emerged. In the first model, an amyloid-associated phenotype arises through the loss of a protein’s normal function when it is incorporated into aggregates. The most well-studied examples of loss-of-function amyloid phenotypes are the S. cerevisiae prion proteins (PrPs) Ure2, Swi1, Cyc8, Mot3, Sfp1 and Sup35, whose amyloid states phenocopy deletions or mutations in these factors [1] . In the second model, an amyloid-associated phenotype arises through the gain of a novel function when a protein is incorporated into aggregates. The most widely studied gain-of-function phenotype is the toxicity associated with mammalian proteins implicated in neurodegenerative diseases, such as PrP in Creutzfeldt–Jakob and mad cow diseases, Aβ in Alzheimer’s disease and huntingtin in Huntington’s disease. However, gain-of-function beneficial traits, such as hormone storage, biofilm formation, organelle biogenesis and long-term memory are also associated with the assembly of other proteins into amyloid [1] , [3] , [4] , [5] . Regardless of the model, the protein-based phenotypes were originally believed to emerge once the amyloid accumulated beyond the threshold required to impact normal physiology. However, studies in multiple systems have uncoupled amyloid accumulation from its phenotypic effects. In mammals, pathogenesis correlates poorly with the accumulation of ataxin-1 (ref. 6 ) or huntingtin [7] inclusions or protease-resistant PrP [8] , [9] , [10] , hallmarks of the amyloid state. Modulation of chaperone expression ameliorates toxicity of polyglutamine-expanded proteins in Drosophila without impacting their accumulation in aggregates [11] , [12] , [13] . And finally, in Caenorhabditis elegans , depletion of the insulin/insulin-like growth factor-1 receptor DAF-2 suppresses Aβ 1–42 toxicity while promoting the accumulation of high molecular weight aggregates of the peptide [14] . In many of these cases, the manipulations have now been shown to alter the amyloid assembly pathway and to either promote or deplete the accumulation of intermediates, implicating alternative species in the production of these organismal phenotypes [2] , [15] . However, alterations to the assembly pathway could also impact the physical properties of the amyloid that does accumulate and thereby the phenotypic consequences of this process. In this previously unexplored scenario, multiple protein species would contribute to the observed phenotypes, and changes in assembly pathway dynamics would modulate the associated traits by altering the ratios of the contributing species. Here, we experimentally address this possibility for the yeast prion [ PSI + ], the amyloid form of the eukaryotic release factor 3 (eRF3/Sup35) [16] , [17] , [18] . In non-prion [ psi − ] cells, Sup35 is soluble and facilitates translation termination, but in prion [ PSI + ] cells, Sup35 is aggregated and functionally compromised, leading to the readthrough of stop codons [19] , [20] . The severity and toxicity of the [ PSI + ] state were previously thought to reflect the equilibrium between aggregated (non-functional) and soluble (functionally engaged Sup35) (refs 21 , 22 ), but our studies, presented here, now demonstrate that Sup35 amyloid contributes to the level of translation termination activity in [ PSI + ] cells. The functional contribution of these complexes, however, is impacted by their composition and size, and these amyloid-associated effects are sufficient to explain fluctuations in the prion phenotype. Aggregated Sup35 interacts with its functional partners Loss-of-function mutations in Sup35 phenocopy the translation termination defect observed in a [ PSI + ] strain [23] . However, the existence of gain-of-function beneficial amyloids indicates that amyloid assembly is not incompatible with biochemical activity and raises the possibility that aggregated Sup35 continues to function in its prion conformation. Several previous observations support this hypothesis. First, the Sup35 carboxy-terminal GTPase domain remains accessible on the surface of amyloid fibres in vitro [24] , [25] . Second, Sup35 retains the ability to hydrolyse GTP in its aggregated form in vitro [26] . Third, proteins fused to the amino-terminal Sup35 prion-determining domain (PrD), such as green fluorescent protein (GFP) and luciferase, retain their activity when incorporated into Sup35 aggregates in [ PSI + ] cells [19] , suggesting that conformational conversion is restricted to the domain required for amyloid formation. Nevertheless, Sup35 must still bind to its functional partner Sup45, the eukaryotic release factor 1, and the ribosome to facilitate translation termination [27] , and its ability to engage in these interactions could be compromised by aggregation [24] . As a first step towards determining the contribution of aggregated Sup35 to termination activity in a [ PSI + ] strain, we assessed its ability to associate with Sup45 and the ribosome. Previous studies disagree on whether aggregated Sup35 binds to Sup45 (refs 28 , 29 ) or not [19] , [30] , [31] in [ PSI + ] cells, but in these studies, binding was assessed indirectly by the prion-dependent fractionation of Sup45 to the aggregate-containing pellet following high-speed centrifugation of yeast lysates. A direct assessment of Sup45 association with Sup35 aggregates, however, is complicated by the fact that [ PSI + ] cells contain a mixture of both soluble and aggregated Sup35 [19] , [20] . To circumvent this difficulty, we developed a system to specifically monitor association of functional partners with Sup35 aggregates based on the ability of the PrD to co-aggregate with full-length Sup35 [19] , [20] , [32] . As expected, the Sup35 PrD tagged with an HA epitope (PrD-HA), associated with full-length Sup35 in a [ PSI + ] but not a [ psi − ] strain, as assessed by immunocapture ( Fig. 1a ), demonstrating the ability of this approach to specifically recover aggregated Sup35. Using this PrD-HA system, Sup45 was also specifically co-immunocaptured (IC) with PrD-HA from [ PSI + ] but not [ psi − ] lysates ( Fig. 1a ). Thus, aggregated Sup35 retains its ability to associate with Sup45 in a [ PSI + ] strain. 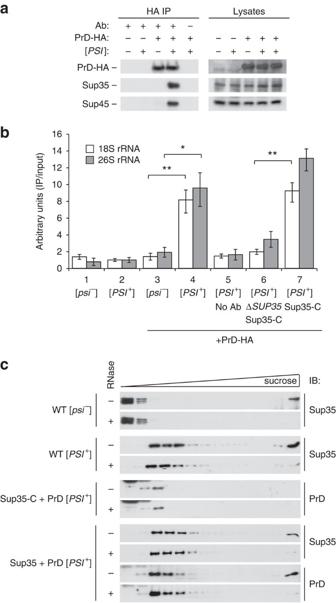Figure 1: Aggregated Sup35 associates with Sup45 and the ribosome in [PSI+] cells. (a) PrD-HA expressed in haploid [PSI+] (+) or [psi−] (−) yeast strains was IC from lysates (Ab, +) in comparison with a reaction lacking specific antiserum (Ab, −), and the isolated complexes were analysed by SDS–PAGE and IB for PrD, Sup35 and Sup45. Total protein in the cell lysates was analysed in parallel to ensure equivalent expression and extraction. (b) Following PrD-HA IC as ina, the presence of ribosomal subunits was assessed by quantitative RT–PCR (qRT–PCR) using primers specific for either 18S or 26S rRNAs. All strains express untagged full-length Sup35 except lane 6, which contains a Sup35 deletion. Lanes 6 and 7 also express the GTPase domain of Sup35 (Sup35-C). The data represent the average of at least three independent experiments, and the error bars represent s.e.m.; *P=0.013; **P≤0.004 by unpaired Student’st-test. (c) Sucrose density gradients were used to fractionate lysates isolated from WT [psi−] or [PSI+] strains and from [PSI+] strains expressing the PrD in the presence of Sup35-C or full-length Sup35. The lysates were either untreated (−) or treated with RNase (+) before fractionation. Following centrifugation, 14 fractions including the pellet were collected and analysed by IB for Sup35 or the PrD. Figure 1: Aggregated Sup35 associates with Sup45 and the ribosome in [ PSI + ] cells. ( a ) PrD-HA expressed in haploid [ PSI + ] (+) or [ psi − ] (−) yeast strains was IC from lysates (Ab, +) in comparison with a reaction lacking specific antiserum (Ab, −), and the isolated complexes were analysed by SDS–PAGE and IB for PrD, Sup35 and Sup45. Total protein in the cell lysates was analysed in parallel to ensure equivalent expression and extraction. ( b ) Following PrD-HA IC as in a , the presence of ribosomal subunits was assessed by quantitative RT–PCR (qRT–PCR) using primers specific for either 18S or 26S rRNAs. All strains express untagged full-length Sup35 except lane 6, which contains a Sup35 deletion. Lanes 6 and 7 also express the GTPase domain of Sup35 (Sup35-C). The data represent the average of at least three independent experiments, and the error bars represent s.e.m. ; * P =0.013; ** P ≤0.004 by unpaired Student’s t -test. ( c ) Sucrose density gradients were used to fractionate lysates isolated from WT [ psi − ] or [ PSI + ] strains and from [ PSI + ] strains expressing the PrD in the presence of Sup35-C or full-length Sup35. The lysates were either untreated (−) or treated with RNase (+) before fractionation. Following centrifugation, 14 fractions including the pellet were collected and analysed by IB for Sup35 or the PrD. Full size image Ribosomes were also specifically co-IC with PrD-HA from a [ PSI + ] but not a [ psi − ] lysate, as assessed by reverse transcriptase PCR (RT–PCR) of ribosomal RNA (rRNA) ( Fig. 1b ), suggesting an association with aggregated Sup35 as well. Because ribosomes are in excess to Sup35 in vivo [33] , [34] , we performed additional experiments to confirm the specificity of this interaction. Notably, PrD-HA immunocapture was unable to recover ribosomes in a strain whose only functional source of Sup35 activity was the Sup35 catalytic domain (Sup35-C), which cannot interact with prion aggregates ( Fig. 1b , lane 6) [32] However, PrD-HA immunocapture recovered ribosomes in the presence of full-length Sup35 ( Fig. 1b , compare lanes 4 and 7 with lane 6). Because full-length Sup35 binds to PrD-HA only in a [ PSI + ] strain ( Fig. 1a ), the dependence of the PrD-HA/ribosome interaction on this protein indicates that prion aggregates interact with ribosomes. As a further test of this interaction, we examined the dependence of the PrD-HA/ribosome interaction on full-length Sup35 through biochemical fractionation on sucrose gradients. Under these conditions, Sup35 fractionated to the top of the gradient from [ psi − ] lysates and to intermediate fractions from [ PSI + ] lysates ( Fig. 1c ). These migration patterns were not perturbed by RNase treatment ( Fig. 1c ), which destroyed rRNA ( Supplementary Fig. 1 ), indicating that they reflect prion-dependent differences in Sup35 assembly rather than ribosome association. In addition to these Sup35 pools, a fraction of Sup35 was also recovered in the pellet from both [ PSI + ] and [ psi − ] lysates ( Fig. 1c ). RNase treatment of the lysates led to the loss of pelletable Sup35 ( Fig. 1c ), suggesting that this fraction reflects ribosome-engaged Sup35. Notably, the PrD alone did not fractionate to the pellet, but it did so in the presence of full-length Sup35 and intact rRNA in a [ PSI + ] lysate ( Fig. 1c , compare Sup35-C+PrD with Sup35+PrD). Thus, this pelleted material contains prion aggregates that are likely engaged with ribosomes in vivo . Aggregated Sup35 functions in translation termination These observations, together, indicate that aggregated Sup35 interacts with its functional partners in [ PSI + ] cells. But, do these interactions contribute to translation termination activity in [ PSI + ] cells? To begin to answer this question, we first established the relationship between Sup35 abundance and activity in vivo . To do so, we expressed Sup35 from a doxycycline-repressible promoter as the sole source of the protein in a [ psi − ] strain and assessed stop-codon readthrough using a glutathione- S -transferase (GST)(UGA)DsRedNLS reporter as a function of Sup35 abundance [35] . In this system, Sup35 activity was present in excess, as termination fidelity was maintained until the level of the protein fell to ~40% with increasing concentrations of doxycycline ( Fig. 2a ). Below this threshold, there was a near linear increase in stop-codon readthrough, consistent with a limitation in the availability of Sup35 ( Fig. 2a ). In a wild-type (WT) [ psi − ] strain, Sup35 was fully soluble, and stop-codon readthrough was barely detectible ( Fig. 2a ). This combination of parameters placed the [ psi − ] state directly on the dose–response curve generated for Sup35 activity by doxycycline titration ( Fig. 2a ). In contrast, only ~10% of Sup35 protein was soluble in a WT [ PSI + ] strain, which exhibited a nearly 30-fold increase in stop-codon readthrough relative to a WT [ psi − ] strain ( Fig. 2a ). However, the level of stop-codon readthrough observed in the [ PSI + ] strain was significantly reduced in comparison with the level predicted for ~10% soluble Sup35 by the dose–response curve ( Fig. 2a ). These findings imply that aggregated Sup35 makes an appreciable contribution to termination activity in a [ PSI + ] strain. 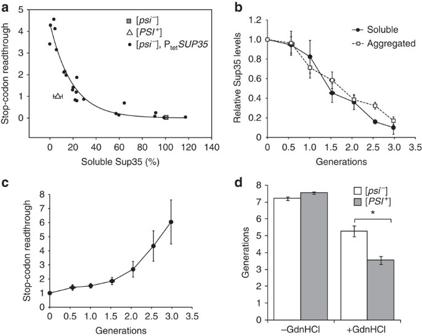Figure 2: Aggregated Sup35 contributes translation termination activity to [PSI+] cells. (a) The levels of soluble Sup35 relative to a WT [psi−] strain and stop-codon readthrough relative to WT [PSI+] strain were determined in lysates from WT [psi−] (grey square), WT [PSI+] (white triangle) and [psi−] strains expressing Sup35 from a doxycycline-repressible promoter (Ptet; black circles). These strains also expressed a reporter for stop-codon readthrough (GST(UGA)DsRedNLS). The levels of Sup35 and GST were determined by quantitative IB. Error bars represent s.d.;n=6. (b) The relative levels of soluble (black circles) and aggregated (white squares) Sup35 in a Ptet-SUP35[PSI+] strain were determined at the indicated generations following doxycycline-induced repression of Sup35 synthesis by quantitative IB. Error bars represent s.e.m.;n=3. (c) The relative level of stop-codon readthrough of GST(UGA)DsRedNLS in a Ptet-SUP35[PSI+] strain was determined by analysis of lysates by quantitative IB for GST at various times after addition of doxycycline. Error bars represent s.e.m.;n=3. (d) [PSI+] (grey) and [psi−] (white) zygotes with repressed Sup35 synthesis were analysed by microscopy to determine the number of generations supported by the existing pool of Sup35 in the absence (−) and presence (+) of guanidine hydrochloride (GdnHCl). Error bars represent s.e.m.;n≥ 20; *P=0.0001 by unpaired Student’st-test. Figure 2: Aggregated Sup35 contributes translation termination activity to [ PSI + ] cells. ( a ) The levels of soluble Sup35 relative to a WT [ psi − ] strain and stop-codon readthrough relative to WT [ PSI + ] strain were determined in lysates from WT [ psi − ] (grey square), WT [ PSI + ] (white triangle) and [ psi − ] strains expressing Sup35 from a doxycycline-repressible promoter (P tet ; black circles). These strains also expressed a reporter for stop-codon readthrough (GST(UGA)DsRedNLS). The levels of Sup35 and GST were determined by quantitative IB. Error bars represent s.d. ; n =6. ( b ) The relative levels of soluble (black circles) and aggregated (white squares) Sup35 in a P tet - SUP35 [ PSI + ] strain were determined at the indicated generations following doxycycline-induced repression of Sup35 synthesis by quantitative IB. Error bars represent s.e.m. ; n =3. ( c ) The relative level of stop-codon readthrough of GST(UGA)DsRedNLS in a P tet - SUP35 [ PSI + ] strain was determined by analysis of lysates by quantitative IB for GST at various times after addition of doxycycline. Error bars represent s.e.m. ; n =3. ( d ) [ PSI + ] (grey) and [ psi − ] (white) zygotes with repressed Sup35 synthesis were analysed by microscopy to determine the number of generations supported by the existing pool of Sup35 in the absence (−) and presence (+) of guanidine hydrochloride (GdnHCl). Error bars represent s.e.m. ; n ≥ 20; * P =0.0001 by unpaired Student’s t -test. Full size image If both aggregated and soluble Sup35 do contribute to termination activity, we would expect that depletion of Sup35 would lead to an increase in stop-codon readthrough only when the total functional pool of Sup35 (that is, both aggregated and soluble forms of the protein) became limiting. However, if only soluble Sup35 contributed to termination activity in [ PSI + ] cells, we would predict that depletion of Sup35 would lead directly to an increase in stop-codon readthrough because the level of soluble Sup35 in a [ PSI + ] strain is already below the threshold for faithful termination ( Fig. 2a ). To test this idea, we expressed Sup35 from a doxycycline-repressible promoter as the sole source of the protein in a [ PSI + ] strain. As expected, addition of doxycycline led to a decrease in the steady-state level of Sup35 over time ( Fig. 2b ). Notably, this inhibition of Sup35 synthesis led to a parallel decrease in both the soluble and aggregated pools of Sup35, indicating that the equilibrium between the two forms of the protein was not perturbed ( Fig. 2b ). On depletion of Sup35, stop-codon readthrough increased beyond the level observed in a [ PSI + ] strain, but an appreciable increase was only observed after 1.5 generations ( Fig. 2c ). During this time, ~50% of Sup35 was depleted ( Fig. 2b ), which was consistent with the threshold for the increase in stop-codon readthrough that we determined in a [ psi − ] strain ( Fig. 2a ). Thus, aggregated Sup35 must contribute to termination activity in a [ PSI + ] strain. As a complementary approach, we also assessed strain viability on Sup35 depletion, as the activity of this protein is essential [23] . If soluble Sup35 was the only active form of the protein, we would predict viability to be lost earlier following the depletion of Sup35 in a [ PSI + ] strain, which accumulates only ~10% soluble Sup35 at steady state ( Fig. 2a ), than in a [ psi − ] strain, where Sup35 is fully soluble ( Fig. 2a ). To test this possibility, we expressed Sup35 from the cell type-specific promoters P MFA1 and P MFα1 in MATa and MAT α strains, respectively, and mated these strains together to repress new Sup35 synthesis [35] . We then determined the number of generations supported by the existing pool of Sup35 in [ PSI + ] and [ psi − ] strains by microscopy. Using this system, a [ psi − ] strain persisted for an average of seven generations after repression of Sup35 synthesis. Remarkably, the viability of the [ PSI + ] strain was similar ( Fig. 2d ), consistent with our observations that aggregated protein must contribute to the overall level of Sup35 activity in [ PSI + ] cells ( Fig. 2a,c ). If this scenario is indeed the case, conditions that reduce the transmission of Sup35 aggregates to daughter cells, such as treatment with a low level of guanidine HCl (GdnHCl) [36] , [37] , should strongly compromise viability of the [ PSI + ] strain by promoting the more rapid depletion of the existing protein. For the [ psi − ] strain, viability was reduced to an average of five generations in the presence of GdnHCl, presumably reflecting the mild toxicity of the treatment ( Fig. 2d ) [38] . However, viability was more severely reduced to an average of 3.5 generations in the [ PSI + ] strain on GdnHCl treatment, consistent with a role for aggregated protein in the overall level of Sup35 activity in a [ PSI + ] strain. [ PSI + ] toxicity does not correlate with soluble Sup35 loss How does this discovery of aggregate-associated activity impact our mechanistic understanding of the [ PSI + ] phenotype? To address this question, we considered prion toxicity. Under normal laboratory growth conditions, some [ PSI + ] isolates are not detrimental to yeast [39] , [40] , but these isolates become toxic on overexpression of either the PrD or full-length Sup35 [22] , [31] , [41] , [42] , [43] . This toxicity has been linked to the availability of either Sup35 or Sup45, respectively [31] . In the case of PrD overexpression, a previous study proposed that toxicity resulted from the depletion of the small soluble pool of full-length Sup35 in a [ PSI + ] strain through its incorporation into aggregates by mass action [31] . However, the creation of new templates to accept this soluble protein is dependent on the activity of the molecular chaperone Hsp104 and its co-chaperones Hsp70 (Ssa1/2) and Sis1, which together fragment larger aggregates into smaller complexes [1] . This limitation, based on chaperone availability, may restrict the predicted shift in equilibrium towards the aggregate state [44] . To resolve the mechanism of toxicity associated with Sup35 overexpression in a [ PSI + ] strain, we first determined the effect of PrD overexpression on the level of soluble full-length Sup35. Integration of a plasmid expressing the PrD ~1.3-fold ( Supplementary Fig. 2 ) into a [ PSI + ] strain did not reduce the level of soluble full-length Sup35 in comparison with the parent strain ( Fig. 3a ). To assess the effects of high-copy overexpression of the PrD on the accumulation of soluble Sup35, we constructed a [ PSI + ] yeast strain expressing full-length Sup35 from its own promoter and Sup35-C from a doxycycline-repressible promoter. Sup35-C lacks the PrD, is incapable of incorporating into prion aggregates and suppresses the toxicity of overexpressed PrD [31] . We then transformed this strain with a PrD-encoding high-copy plasmid, which leads to ~10-fold overexpression of the PrD on medium lacking uracil or ~100-fold overexpression of the PrD on medium lacking leucine [31] . On medium lacking uracil, the levels of soluble full-length Sup35 decreased only approximately twofold relative to a vector control ( Fig. 3b ). This modest decrease was similar on medium lacking leucine despite the 10-fold increase in Sup35 expression relative to the medium lacking uracil ( Fig. 3b ). Thus, the equilibrium between soluble and aggregated protein is limited by factors beyond Sup35 concentration. 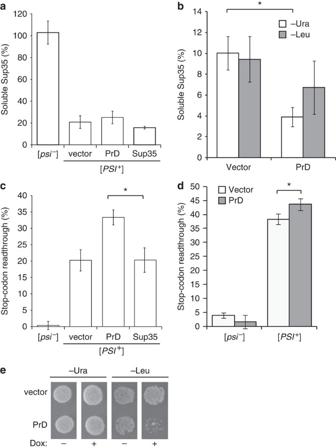Figure 3: The severity and toxicity of the [PSI+] state cannot be explained by fluctuations in the level of soluble Sup35. (a) The levels of soluble Sup35 were determined in lysates from WT [psi−] and [PSI+] strains and from [PSI+] strains expressing full-length Sup35 from Ptetat ~1.5-fold the WT level (Sup35) or the PrD from PSUP35(PrD) by quantitative IB for Sup35. All strains also expressed the stop-codon readthrough reporter GST(UGA)DsRedNLS. Error bars represent s.e.m.;n≥3. (b) Strains expressing full-length Sup35 from PSUP35and Sup35-C from Ptetwere transformed with either vector or a high-copy plasmid that overexpresses the PrD ~10-fold on medium lacking uracil (−Ura) or ~100-fold on medium lacking leucine (−Leu). The levels of soluble Sup35 under these conditions were determined in lysates by quantitative IB. Error bars represent s.e.m.;n≥5; *P=0.004 by unpaired Student’st-test. (c) Stop-codon readthrough was determined in lysates from the strains described inaby quantitative IB for GST. Error bars represent s.e.m.;n≥3; *P=0.017 by unpaired Student’st-test. (d) Stop-codon readthrough was determined as inein lysates from the strains described inb. Strains were grown in medium lacking uracil (−Ura) in the presence of doxycycline to repress expression of Sup35-C. Error bars represent s.e.m.;n≥3; *P=0.01 by unpaired Student’st-test. The differences in levels of stop-codon readthrough incanddrepresent the different baselines in richcand minimaldmedium. (e) The strains described inbwere plated on medium lacking uracil (−Ura) or lacking leucine (−Leu) in the absence (−) or presence (+) of doxycycline to repress Sup35-C expression and assess toxicity of overexpressed Sup35. Figure 3: The severity and toxicity of the [ PSI + ] state cannot be explained by fluctuations in the level of soluble Sup35. ( a ) The levels of soluble Sup35 were determined in lysates from WT [ psi − ] and [ PSI + ] strains and from [ PSI + ] strains expressing full-length Sup35 from P tet at ~1.5-fold the WT level (Sup35) or the PrD from P SUP35 (PrD) by quantitative IB for Sup35. All strains also expressed the stop-codon readthrough reporter GST(UGA)DsRedNLS. Error bars represent s.e.m. ; n ≥3. ( b ) Strains expressing full-length Sup35 from P SUP35 and Sup35-C from P tet were transformed with either vector or a high-copy plasmid that overexpresses the PrD ~10-fold on medium lacking uracil (−Ura) or ~100-fold on medium lacking leucine (−Leu). The levels of soluble Sup35 under these conditions were determined in lysates by quantitative IB. Error bars represent s.e.m. ; n ≥5; * P =0.004 by unpaired Student’s t -test. ( c ) Stop-codon readthrough was determined in lysates from the strains described in a by quantitative IB for GST. Error bars represent s.e.m. ; n ≥3; * P =0.017 by unpaired Student’s t -test. ( d ) Stop-codon readthrough was determined as in e in lysates from the strains described in b . Strains were grown in medium lacking uracil (−Ura) in the presence of doxycycline to repress expression of Sup35-C. Error bars represent s.e.m. ; n ≥3; * P =0.01 by unpaired Student’s t -test. The differences in levels of stop-codon readthrough in c and d represent the different baselines in rich c and minimal d medium. ( e ) The strains described in b were plated on medium lacking uracil (−Ura) or lacking leucine (−Leu) in the absence (−) or presence (+) of doxycycline to repress Sup35-C expression and assess toxicity of overexpressed Sup35. Full size image Exploiting the different effects of these three levels of PrD expression, we next determined the relationship between the availability of soluble, full-length Sup35 and prion phenotypes by assessing stop-codon readthrough and toxicity in these strains. For the high-copy condition, doxycycline was added to the growth medium to repress expression of Sup35-C and allow detection of these phenotypes. Although only high-copy PrD expression affected the level of soluble full-length Sup35 ( Fig. 3a,b ), both single ( Fig. 3c ) and high-copy ( Fig. 3d ) overexpression (assessed on medium lacking uracil) of the PrD led to an increase in stop-codon readthrough. In the case of toxicity, growth impairment was only observed with the highest level of PrD overexpression attained in medium lacking leucine ( Fig. 3e ), although growth on medium lacking either uracil or leucine led to a similar reduction in the accumulation of soluble full-length Sup35 ( Fig. 3b ). Thus, these observations reveal additional discordance between Sup35 solubility and activity in a [ PSI + ] strain and, together with the finding that Sup35 aggregates contribute to the overall level of termination activity in a [ PSI + ] strain ( Fig. 2a ), indicate that previously unanticipated factors contribute to the severity of prion phenotypes. Sup35 aggregate composition and size impacts activity What molecular events might explain these disconnects between Sup35 solubility and activity? In addition to the modest changes in the accumulation of soluble Sup35 that we observed on PrD overexpression, increasing the synthesis rate of the PrPs will also increase the size of aggregates, due to the chaperone-limited fragmentation reaction [44] . This increase in aggregate size could also impact the contribution that Sup35 aggregates make to the overall level of translation termination activity in [ PSI + ] cells. Our first indication that this hypothesis might be valid was the disparate behaviour of PrD expression from that of mild overexpression of full-length Sup35 in a WT [ PSI + ] strain. Notably, modest (~1.5-fold, Supplementary Fig. 2 ) overexpression of full-length Sup35 from a doxycycline-repressible promoter did not lead to the increase in stop-codon readthrough observed in cells expressing a similar level of the PrD ( Fig. 3c ). Given the fact that neither condition perturbed the equilibrium between soluble and aggregated full-length Sup35 ( Fig. 3a ), the most parsimonious interpretation of this observation is that the incorporation of the PrD into aggregates of full-length Sup35 diminishes their activities by altering their composition. To further explore the possibility that overexpression of the PrD reduces aggregate activity, we next assessed their ribosome engagement in the presence of high-copy PrD. Lysates from strains expressing different amounts of the PrD, as well as from control strains, were fractionated on sucrose gradients, and the amount of full-length Sup35 in the ribosome-containing pellet was determined. Similar amounts of pelleted Sup35 were observed in lysates regardless of whether these cells overexpressed the PrD by ~10-fold or not ( Fig. 4a , −Ura). In contrast, the partitioning of Sup35 to the pellet was reduced approximately fourfold when lysates from cells overexpressing the PrD by ~100-fold were analysed ( Fig. 4a , −Leu). Because only the strong overexpression of the PrD is toxic to cells ( Fig. 3e ), these results indicate that prion toxicity correlates with a depletion of ribosome-engaged, aggregated Sup35. 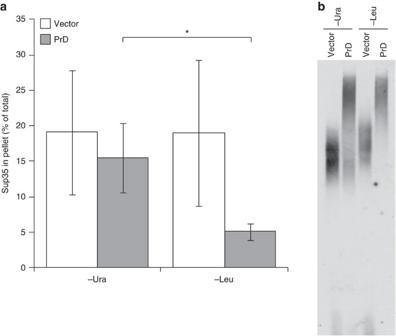Figure 4: The toxicity associated with PrD overexpression correlates with a depletion of a subclass of Sup35 aggregates. (a) Lysates from [PSI+] strains overexpressing the PrD as described inFig. 3bthat were grown in medium lacking either uracil (−Ura) or leucine (−Leu) were fractionated on sucrose gradients and analysed by quantitative IB for Sup35 as described inFig. 1c. The percentage of Sup35 in the pellet was determined relative to the total amount of Sup35 distributed across the gradient. Error bars represent s.e.m.;n≥5; *P=0.017 by unpaired Student’st-test. (b) Lysates from strains described inawere grown in medium lacking uracil (−Ura) or leucine (−Leu) and were analysed by semi-denaturating detergent agarose gel electrophoresis and IB for Sup35. Lysates were normalized for Sup35 expression before loading to allow comparisons of aggregate size. Figure 4: The toxicity associated with PrD overexpression correlates with a depletion of a subclass of Sup35 aggregates. ( a ) Lysates from [ PSI + ] strains overexpressing the PrD as described in Fig. 3b that were grown in medium lacking either uracil (−Ura) or leucine (−Leu) were fractionated on sucrose gradients and analysed by quantitative IB for Sup35 as described in Fig. 1c . The percentage of Sup35 in the pellet was determined relative to the total amount of Sup35 distributed across the gradient. Error bars represent s.e.m. ; n ≥5; * P =0.017 by unpaired Student’s t -test. ( b ) Lysates from strains described in a were grown in medium lacking uracil (−Ura) or leucine (−Leu) and were analysed by semi-denaturating detergent agarose gel electrophoresis and IB for Sup35. Lysates were normalized for Sup35 expression before loading to allow comparisons of aggregate size. Full size image PrD overexpression, like that of full-length Sup35, is also predicted to increase the size of Sup35 aggregates in vivo due to the enzyme limitation of the fragmentation reaction [44] . In vivo , Sup35 aggregates are composed of SDS-resistant polymers that assemble together into a larger native complex, which scales with the size of the polymers [45] . With a single extra copy of the PrD expressed from the SUP35 promoter, the migration of aggregates on semi-denaturing detergent agarose gels, which preserve the core polymers but not native aggregates, was similar to those isolated from a WT strain ( Supplementary Fig. 3 ), suggesting that the increase in stop-codon readthrough associated with this level of PrD expression results from a change in aggregate composition rather than size. However, PrD overexpression from the high-copy plasmid had strong effects on Sup35 aggregate size in a [ PSI + ] strain. When PrD overexpression was induced ~10-fold by growth in medium lacking uracil, some SDS-resistant aggregates remained in the range observed in lysates from the vector control strain ( Fig. 4b ). However, these species were completely depleted in lysates from cells grown in medium lacking leucine in which the PrD is overexpressed by ~100-fold ( Fig. 4b ) Thus, toxicity correlates with both the depletion of ribosome-engaged Sup35 aggregates and an increase in aggregate size. To separate the contributions of aggregate composition and size to their activity in vivo , we took advantage of the fact that Sup35 assembles into aggregates of different sizes based on its conformation and the state of cellular proteostasis. For example, Sup35 can adopt a spectrum of conformations that lead to distinct phenotypic states, characterized by the level of stop-codon readthrough [22] , [46] . Conformations associated with a ‘weak’ phenotype assemble into aggregates of higher thermodynamic stability, increased size and decreased transmissibility relative to conformations associated with a ‘strong’ phenotype ( Fig. 5a ) [21] , [44] , [45] . Moreover, deletion of the N-terminal acetyltransferase NatA reduces the size of Sup35 aggregates ( Fig. 5a ) without altering the equilibrium between aggregated and soluble protein through a complex pathway [47] , and these changes result in a reversal of the translation termination defect in [ PSI + ] cells [47] , [48] . Using this panel of strains expressing a single copy of PrD-HA, we correlated Sup35 aggregate size with translation termination activity and ribosome association. 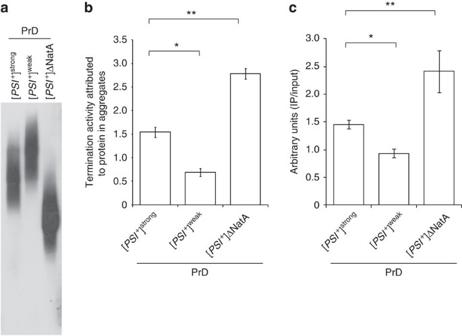Figure 5: Sup35 aggregate size correlates inversely with aggregate activity and association with ribosomes. (a) Lysates from [PSI+]strong, [PSI+]weakand [PSI+] ΔNatA strains, each expressing PrD and GST(UGA)DsRedNLS, were analysed by semi-denaturating detergent agarose gel electrophoresis and IB for Sup35. (b) Termination activity attributed to aggregates was determined in lysates isolated from the strains described inaby quantitative IB for GST. Error bars represent s.e.m.;n=3; *P=0.0031 and **P=0.0012 by unpaired Student’st-test. (c) Lysates isolated from the strains described inawere IC as described inFig. 1bfor 18S rRNA. Error bars represent s.e.m.;n=3; *P=0.001 and **P=0.0004 by unpaired Student’st-test. Figure 5: Sup35 aggregate size correlates inversely with aggregate activity and association with ribosomes. ( a ) Lysates from [ PSI + ] strong , [ PSI + ] weak and [ PSI + ] ΔNatA strains, each expressing PrD and GST(UGA)DsRedNLS, were analysed by semi-denaturating detergent agarose gel electrophoresis and IB for Sup35. ( b ) Termination activity attributed to aggregates was determined in lysates isolated from the strains described in a by quantitative IB for GST. Error bars represent s.e.m. ; n =3; * P =0.0031 and ** P =0.0012 by unpaired Student’s t -test. ( c ) Lysates isolated from the strains described in a were IC as described in Fig. 1b for 18S rRNA. Error bars represent s.e.m. ; n =3; * P =0.001 and ** P =0.0004 by unpaired Student’s t -test. Full size image Taking into account differences in the equilibrium between aggregated and soluble Sup35 using our dose–response curve ( Fig. 2a ), we observed an inverse correlation between aggregate size and activity in translation termination. For the [ PSI + ] strong strain, which accumulated Sup35 aggregates of intermediate size ( Fig. 5a ), we observed an intermediate level of aggregate-associated translation termination activity ( Fig. 5b ). Relative to the [ PSI + ] strong strain, the increased Sup35 aggregate size observed in a [ PSI + ] weak strain correlated with a decrease in aggregate-associated activity, and the decreased Sup35 aggregate size observed in a [ PSI + ] strong ΔNatA strain correlated with an increase in aggregate-associated activity ( Fig. 5b ). Following immunocapture of PrD-HA and analysis of rRNA by RT–PCR, we also noted an inverse correlation with size. The intermediate size aggregates isolated from the [ PSI + ] strong strain captured an intermediate level of ribosomes; the larger aggregates isolated from the [ PSI + ] weak strain captured a lower level of ribosomes, and the smaller aggregates isolated from the [ PSI + ] strong ΔNatA strain captured a higher level of ribosomes ( Fig. 5c ). Thus, beyond changes in aggregate composition, our observations indicate that smaller Sup35 aggregates engage the ribosome more efficiently and contribute more termination activity to the cell than their larger counterparts. To develop a more quantitative relationship between Sup35 aggregate size and activity, we took advantage of our previously developed mathematical model of prion propagation [44] . Our previous studies accurately captured the [ PSI + ] strong and [ PSI + ] weak states, and we used the same model but with a 3-fold increase in the [ PSI + ] strong fragmentation rate to capture the [ PSI + ] strong ΔNatA state, which has an increased accumulation of Hsp104 [47] . Using these parameters, we numerically generated aggregate size distributions for the three strains ( Fig. 6a ), and these outputs accurately recapitulate our experimental observations ( Fig. 5a ). Using these distributions, we explored three models to explain the activity of Sup35 aggregates relative to their size in a [ PSI + ] strain: (1) a linear increase in activity with size, (2) no change in activity with size and (3) a power decrease in activity with size. 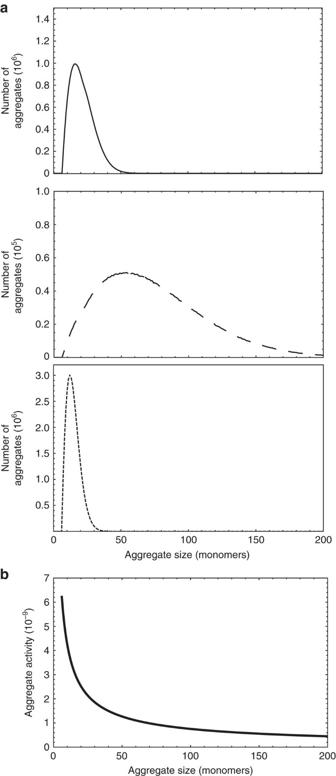Figure 6: Mathematical modelling supports an inverse correlation between Sup35 aggregate size and activity. (a) Aggregate size distributions for [PSI+]strong(solid) [PSI+]weak(dashed), and [PSI+] ΔNatA (dotted) resulting from stochastic simulations of a mathematical model for prion propagation. (b) The relationship between aggregate activity and size corresponding to model 3 (power decrease in activity with size) forβ=0.25 (see text for details). Figure 6: Mathematical modelling supports an inverse correlation between Sup35 aggregate size and activity. ( a ) Aggregate size distributions for [ PSI + ] strong (solid) [ PSI + ] weak (dashed), and [ PSI + ] ΔNatA (dotted) resulting from stochastic simulations of a mathematical model for prion propagation. ( b ) The relationship between aggregate activity and size corresponding to model 3 (power decrease in activity with size) for β =0.25 (see text for details). Full size image We next calculated the least squares solution that most accurately explains the empirically determined aggregate activities ( Fig. 5b ) and the dose–response curve for the corresponding level of soluble Sup35 present ( Fig. 2a ) for each of the model formulations. To compare the fits, we calculated the residual sum of the least squares errors for each model and the Akaike Information Criterion (AIC) ( Table 1 ). AIC is a common model selection test, which considers both the agreement of a statistical model to a given data set and the complexity (number of parameters) of the model. When comparing between models, the model with the lowest AIC is preferred. For model 3, we explored a range of powers ( β ), and selected a solution of 0.276, the minimum of the residual sum of the least squares errors, as the optimum value ( Supplementary Fig. 4 ). (Note, a linear decrease in aggregate activity with size is represented by the condition β =−1.) As expected, based on the inverse correlation between aggregate size and activity that we measured empirically ( Fig. 5b ), the first model (activity increases linearly with size) has the largest residual sum of least squares errors; the second model (no size dependence of activity) has an intermediate residual sum of least squares errors and the third model (activity decreases with size) has the lowest residual sum of least squares errors overall ( Table 1 ). By comparing the ratio of the residual sum of least squares errors, model 3 outperforms model 2 by ~27-fold and model 1 by ~578-fold and, correspondingly, exhibits the lowest AIC of the models ( Table 1 ). Our computational modelling, therefore, reveals an exponential decrease in Sup35 aggregate activity with size ( Fig. 6b ) as the most robust explanation for the phenotypic variability of these states. This model, in contrast to the others, also uniquely explains the observed threshold effect, in which a 10-fold increase in expression of Sup35 converts a completely benign state into a strictly toxic one ( Fig. 3e ), by linking a modest change in aggregate size ( Figs 4b , 5a ) to a drastic reduction in activity ( Fig. 5b ). Thus, amyloid heterogeneity plays an essential role in the determination of protein-only phenotypes. Table 1 Analysis of aggregate activity models. Full size table Loss-of-function yeast prion phenotypes are, at first glance, inconsistent with many previous studies that directly analysed the effects of conformational conversion and assembly on enzymatic activity. For example, diverse proteins, such as GFP, luciferase, carbonic anhydrase III, GST and barnase retain their activities when fused to the PrD of either Sup35 (ref. 19 ) or another yeast PrPs Ure2 and aggregated in [ PSI + ] or [ URE3 ] strains, respectively [49] , and Ure2 retains its native glutathione peroxidase activity in its fibrillar form [50] . However, these enzymes have either intrinsic activity or act on small diffusible substrates, raising the possibility that the loss-of-function prion phenotypes arise from steric occlusion of essential interactions in the aggregate form [24] , [49] . Following from this model, the yeast prion [ PSI + ] was previously thought to confer a translation termination defect through sequestration of Sup35 into amyloid aggregates [19] , [20] . However, our studies reveal that in vivo aggregated Sup35, which exhibits the SDS-resistance of in vitro amyloid fibres [51] , retains interactions with its functional partners Sup45 and ribosomes ( Fig. 1a–c ), consistent with the exposure of its functional C-terminal domain on the surface of amyloid fibres [24] , [25] , and contributes termination activity ( Fig. 2a,c,d ) in [ PSI + ] cells. Thus, the equilibrium between soluble and aggregated Sup35 is insufficient to explain the molecular basis of the [ PSI + ] phenotype in vivo . How does this functional contribution of aggregates impact our understanding of a loss-of-function amyloid phenotype? Within the framework of this refined model, our studies indicate that amyloid aggregates vary in their activities in vivo ( Figs 5a,b and 6b ), and this heterogeneity provides a molecular explanation for previously enigmatic aspects of prion biology in yeast. First, deletion of the N -terminal acetyltransferase NatA reverses the [ PSI + ] phenotype without altering the accumulation of SDS-resistant Sup35 aggregates [47] , [48] . Based on our studies, the smaller complexes that accumulate in this strain ( Fig. 5a ) [47] , [48] have increased translation termination activity ( Fig. 5b ) and ribosome association ( Fig. 5c ), thereby uncoupling Sup35 aggregates from their normal phenotypic effects. Second, benign variants of [ PSI + ] become toxic on overexpression of the PrD [22] , [31] , [41] , [42] , [43] . Based on our observations, this toxicity arises from a decrease in termination activity on PrD incorporation into aggregates of full-length Sup35 at low doses ( Fig. 3c ) and/or to a depletion of smaller, ribosome-engaged aggregates at high doses ( Fig. 4a,b ). Finally, our observations may also provide an explanation for the synthetic lethality of [ PSI + ] with an Hsp104 A503V mutant [52] . While this genetic interaction could reflect a gain-of-function toxicity, expression of Hsp104 A503V in a [ PSI + ] strain increases Sup35 aggregate size, which will decrease the contribution of these complexes to termination activity according to our observations ( Fig. 5b ). Consistent with this interpretation, the toxicity of Hsp104 A503V in a [ PSI + ] strain is suppressed by Sup35-C, suggesting it reflects a Sup35 limitation rather than a gain-of-function phenotype [52] . Thus, variation in the composition and size of SDS-resistant Sup35 aggregates, which impact the engagement of these complexes with its functional partners perhaps through changes in their diffusional properties and/or local concentration effects, is a previously unanticipated contributor to the severity and toxicity of the prion state. In mammals, amyloid toxicity has also been uncoupled from its accumulation in many systems. The general model that has emerged to explain these observations is that intermediates, either on- or off-pathway, that arise during fibrilization are the toxic species [2] , [15] , [53] . Significant experimental support for this toxic intermediate model has been collected in mice, Drosophila , C. elegans , and yeast [6] , [7] , [8] , [9] , [10] , [11] , [12] , [13] , [14] , [54] , but such a model does not exclude potential contributions of other misfolded species, including amyloid [57] , to cellular dysfunction [2] , [53] , [55] , [56] . Detailed temporal studies using several amyloidogenic proteins have uncovered a multi-step pathway of assembly, in which unstructured oligomeric intermediates arise and progress to more structured protofibrils and ultimately to highly ordered fibres [2] , [51] . The relative populations of these misfolded species, which are composed of the same protein, are interconnected and, as such, are all impacted by changes in experimental conditions. Each of these misfolded species will present non-native surfaces to the cellular environment [2] , [56] and may vary in their functional contributions [57] , as we have demonstrated for Sup35 amyloid. Thus, pathogenesis is more likely to reflect the combined effects of this fluctuating population of species, each of which may be associated with a gain and/or loss of function, rather than the appearance of a single toxic species [2] , [56] . Beyond uncovering a functional contribution for aggregates in vivo , our studies highlight the more nuanced, and often underappreciated, role that amyloid heterogeneity plays in defining protein-based traits. Many amyloidogenic proteins can determine a range of phenotypes in vivo based on their aggregation. Especially in the case of prions, this variability is believed to arise from differences in the conformation of the protein [15] , [58] , [59] , which impacts the accumulation of the assembled aggregates by altering the rate of their self-replication [21] , [44] , [60] . Our studies suggest an alternative and, in some cases, likely interconnected possibility that aggregate size and composition also contribute to the phenotypic variability of protein-based traits. Notably, amyloid size has already been linked to prion transmissibility in mammals and in yeast [44] , [60] , and factors that influence the severity and toxicity of protein-based traits, such as overexpression of the protein and differences in the accumulation of proteolytic fragments [2] , [61] , are also likely to alter the physical attributes of aggregates without necessarily changing protein conformation. Thus, amyloid heterogeneity may provide a new window through which protein misfolding disease mechanisms can be viewed. Plasmids All plasmids used in this study are listed in Supplementary Table 1 . SB653 is derived from pRS305 and contains the SUP35 promoter (P SUP35 ) as an Eco RI/ Bam HI fragment followed by PrD-HA 3 as a Pst I/ Sal I fragment subcloned from p316SpSup-HA3-FL [62] . SB782 contains P SUP35 -PrD-HA 3 isolated as a Xho I/ Sac I fragment from SB653 and subcloned into the high-copy leu2-d plasmid pEMBL-yex [32] . SB736 contains the CYC1 promoter (P CYC1 ) as a Sac I/ Xba I fragment and PrD-HA 3 as a BstX I- Cla I fragment in pRS306 [63] . SB531 was generated by inserting the GPD promoter (P GPD ) as a Sac I/ Bam HI fragment, GST-UGA as a Bam HI/ Eco RI fragment and DsRedNLS as an Eco RI/ Xho I fragment into pRS304 [63] . SB581 contains a PrD-GFP fusion as a Bam HI/ Sac I fragment and the SUP35 promoter as an Eco RI/ Bam HI fragment in pRS305 [63] . SB397 contains the SUP35 promoter as an Eco RI/ Bam HI fragment, the PrD as a Bam HI/ Sac II fragment and GFPssrA as a Sac II/ Sac I fragment into pRS306. SB515 contains the MFα1 promoter (P MF α 1 ) as an Ava I/ Bam HI fragment in pFA6a-kanMX4, and SB526 contains the MFA1 promoter (P MFA1 ) as a Bgl II/ Bam HI fragment in pFA6a-kanMX6. Yeast strains All strains are derivatives of 74-D694 [18] and are listed in Supplementary Table 2 . Yeast strains were constructed to ectopically express Sup35, the PrD, or the GST(UGA)DsRedNLS reporter from integrating plasmids ( Supplementary Table 1 ) based on the vectors pRS304, pRS305 or pRS306 [63] . These plasmids were integrated following digestion with Bsu 36I, Ppu MI, or Stu I, respectively. Protein expression was confirmed by immunoblotting (IB) with specific antiserum in all cases. For strains SY2059 and SY2061, the HA 3 epitope was fused to the C terminus of NM–GFP by transformation of a DNA fragment generated by PCR using pFA6a-3HA-kanMX6 [64] as a template and primers JP87 and JP88 ( Supplementary Table 3 ). The promoter and the PrD of Sup35 were replaced at the endogenous locus with the MFA1 promoter by transformation of a PCR fragment generated using SB526 as a template and primers JP8 and 3PMFA1Cterm ( Supplementary Table 3 ). Replacements were selected on complete medium supplemented with G418 and confirmed by PCR. The SUP35 promoter was replaced with P tetO7 by transforming strains with a PCR-generated fragment using pCM225 [65] as a template and primers TRS218 and TRS219 [66] . The SUP35 promoter was replaced with the MFα1 promoter by transforming strains with a PCR fragment using SB515 as a template and primers JP33 and JP34 ( Supplementary Table 3 ). The SUP35 promoter was replaced with the MFA1 promoter by transforming strains with a PCR fragment using SB526 as a template and primers JP30 and JP8 ( Supplementary Table 3 ). SY2076 was generated by mating SY2070 to 74D-694 [ PSI + ] weak (ref. 46 ). SY1170 was generated by mating SY1163 to SY356 [48] . SY2061 was generated by mating SY2050 to SY1170. For all matings, tetrads were dissected by micromanipulation on rich medium, and meiotic progeny were characterized for auxotrophies to allow selection of the appropriate strains. Protein analysis Immunocapture was performed as previously described [67] with the following changes: 25 OD 600 units of cells were collected in early log phase; lysis buffer contained 10 mM MgCl 2 ; all wash steps were performed at 4 °C; lysates were precleared with Protein G Magnetic Beads (New England Biolabs), and immunocapture was performed with anti-HA high affinity rat monoclonal antibody clone 3F10 (Roche Applied Sciences) and Protein G Magnetic Beads (NEB). For RNA isolation, IC samples were treated with proteinase K at 250 μg ml −1 in 50 mM Tris–HCl (pH7.4), 50 mM NaCl, 5 mM EDTA, 0.5% SDS at 42 °C for 1 h. Following proteinase K treatment, phenol:chloroform:isoamyl alcohol (25:24:1) extractions were performed twice followed by ethanol precipitation after the addition of LiCl to 800 mM. Samples were then treated with 4U Turbo DNase (Ambion) for 30 min at 37 °C followed by phenol/chloroform extraction and ethanol precipitation with 100 mM sodium acetate, pH 5.2. Samples were resuspended in DEPC-treated water and analysed by quantitative RT–PCR using SYBR Green One-Step qRT–PCR Kit with ROX (Invitrogen) with 2 mM MgSO 4 and primers JP53 and JP54 for 18S rRNA amplification or JP55 and JP56 for 26S rRNA amplification. Dissociation curves generated a single peak for all qPCR reactions. For sucrose-gradient fractionation, lysates were prepared by glass bead disruption at 4 °C in lysis buffer (40 mM Tris–HCl (pH 7.4), 150 mM KCl, 15 mM MgCl 2 , complete protease inhibitor tablet (Roche Applied Sciences) and 20 U ml −1 rRNAsin (Promega)); rRNAsin was not included in samples to be treated with RNase. Glass beads were separated, and the lysate was precleared for 3 min at 5,900 g at 4 °C. A quantity of 100 μl of the supernatant (200 μg total protein content) was loaded to the top of a 2 ml, 15–60% sucrose gradient made in lysis buffer and centrifuged for 3 h at 31,000 g in a TLS55 swinging bucket rotor using an Optima Max Ultracentrifuge (Beckman). Gradients were separated into thirteen equal fractions by pipetting from the top of each gradient, and the pellet was collected. Samples were analysed by quantitative IB with the appropriate antisera using standard protocols. Samples digested with RNase were incubated with 0.5 μg RNase (Roche) for 15 min at room temperature immediately before loading on the sucrose gradient. RNA visualization was performed by mixing 29 μl of each fraction to generate 7% sucrose, 0.045% Orange G and 1% SDS solution. A quantity of 15 μl of this mix was separated on 0.8% TAE agarose gel with 0.5 μg ml −1 ethidium bromide. Soluble Sup35 fractions were determined by comparing the level of Sup35 entering an SDS–PAGE gel by quantitative IB of lysates treated with 2% SDS at either 53 °C or 100 °C, as previously described [48] . Stop-codon readthrough was determined by analysis of lysates isolated from strains expressing GST(UGA)DsRedNLS by quantitative IB for GST. Stop-codon readthrough was determined as the fraction of GST-DsRedNLS expression relative to total GST (GST and GST-DsRedNLS). The level of stop-codon readthrough attributed to Sup35 aggregates was determined by quantifying the level of soluble Sup35 in the strain by SDS sensitivity as described above, determining the amount of stop-codon readthrough expected for that level of soluble protein based on the dose–response curve in Fig. 2a , and subtracting this level of stop-codon readthrough from the actual level measured using the reporter GST(UGA)DsRedNLS as described above. Activity was calculated by subtracting the stop-codon readthrough attributed to aggregates from unity, and normalizing these levels to the amount of Sup35 in aggregates. For semi-denaturating detergent agarose gel electrophoresis, cells were grown in liquid YPD, collected, washed and mechanically disrupted with glass beads in buffer (50 mM sodium phosphate pH 7.5, 100 mM NaCl, 1 mM DTT, 2 mM PMSF, and 5 μg ml −1 Pepstatin). Following clearing of the lysate at 500 g for 1 min at 4 °C, normalized samples were separated on a 1.5% Tris-glycine agarose gel containing 0.1%SDS, transferred to PVDF membrane and analysed by IB using Sup35-specific antiserum (1:2,000 dilution). Viability assay Zygotes were isolated from the indicated crosses by micromanipulation and were allow to divide at 30 °C until growth ceased. The resulting microcolonies were disrupted using a micromanipulator and individual cells were counted. Generations were extrapolated by calculating the log base 2 of the number of cells. Mathematical modelling Aggregate distributions were computed for the three prion strains using a stochastic simulation model previously presented [44] . Parameter values for the [ PSI + ] strong and [ PSI + ] weak strains were as previously reported [44] . Parameters for the ΔNatA strain were the same for [ PSI + ] strong except the value for fragmentation was increased threefold to account for the elevation of Hsp104 [47] . The associated level of aggregate activity was determined for each strain by first determining the level of activity for the soluble fraction of Sup35. The activity associated with Sup35 for [ psi − ] strains ( Fig. 2a ) was fit using Mathematica's FindFit function to an exponential distribution ( a exp( b ), a =4.33777, b =4.98471). Thus for each simulation, the activity related to the soluble Sup35 was computed using the exponential approximation, and the level of activity attributed to an aggregate was determined using three models: (1) the activity of an aggregate is proportional to the number of monomers ( (2) all aggregates have equal activity ( , where A represents aggregate-associated activity, i represents the number of monomers in an aggregate, and n i represents the number of aggregates of size i ), (3) the activity of an aggregate is proportional to a power ( β ) of the number of monomers ( . In all cases, α represents a proportionality constant between aggregate activity and size distribution. A least squares fit was used to determine the best fitting parameters for each model. Errors in our observations were assumed to be normally distributed with mean zero and the same variance. As such, the AIC values for each model could be determined with the residual sum of squared errors. In these cases AIC= n log(RSS/ n )+2 k +C where RSS is the residual sum of squares, n is the number of data points, k is the number of parameters in the model and C is a constant, which does not contribute to the comparison between models [68] . How to cite this article : Pezza, J. A. et al. Amyloid-associated activity contributes to the severity and toxicity of a prion phenotype. Nat. Commun. 5:4384 doi: 10.1038/ncomms5384 (2014).